MitoNEET-mediated effects on browning of white adipose tissue MitoNEET is an outer mitochondrial membrane protein that, upon overexpression in white adipose tissue (WAT), exerts a positive impact on tissue expansion and whole-body lipid and carbohydrate homeostasis by altering mitochondrial matrix iron metabolism. Here we determine the key transcriptional events in subcutaneous WAT of mice in response to mitoNEET overexpression and a high-fat diet (HFD). Microarray analyses at key points during weight gain upon body weight divergence with wild-type mice demonstrate that mitoNEET-enriched sWAT early on, upregulates a browning signature programme that limits WAT expansion in transgenic mice for a period of up to 12 weeks of HFD. This compensatory browning phenotype is subsequently lost, resulting in rapid WAT expansion and body weight gain. Exposure to thermoneutral temperatures during HFD prompts weight gain significantly earlier. Similar WAT expansion is achieved upon infection with an adeno-associated virus expressing mitoNEET. Collectively, the mitoNEET-enriched fat pads feature a more vascularized, anti-inflammatory and less fibrotic environment. Obesity, now a global epidemic, is associated with a cluster of metabolic disorders such as insulin resistance, type 2 diabetes mellitus (T2DM), hyperlipidemia and hypertension [1] . Intake of high-fat diets (HFD) is a key environmental factor that can profoundly contribute to the development of such metabolic disorders [2] , [3] , [4] . White adipose tissue (WAT) plays a pivotal role in maintaining whole-body energy homeostasis by storing excess energy as triglycerides (TGs) and releasing free fatty acids (FFAs) as a fuel source during energy shortage; processes crucial for proper fuel metabolism. However, during prolonged excessive caloric intake, dramatic expansion of WAT can result in a high mass of dysfunctional, inflamed and fibrotic WAT; in that state, local and whole-body glucose and lipid dysregulation prevails. The protective effect of expandable subcutaneous fat depots during weight gain permits adequate storage of excess calories in the form of TGs to prevent ectopic lipid deposition in non-adipose cells, such as hepatocytes, myocytes and pancreatic β-cells; such lipotoxicity greatly increases the risk of insulin resistance and T2DM [5] , [6] . Therefore, understanding the mechanisms by which subcutaneous (sWAT) expandability is regulated, is of great importance. Particular emphasis is placed on how to sustain healthy non-fibrotic, non-inflamed sWAT expansion during excess nutrient intake, in addition to pushing the maximum capacity for sWAT expansion to higher limits to prevent lipotoxic insults. Under physiological conditions, lipid and glucose homeostasis is largely dependent on fully functional mitochondria, the cellular power houses that generate ATP to sustain cellular function. Mitochondrial dysfunction on the other hand is emerging as a central contributory factor in the development insulin resistance and T2DM [7] , [8] , [9] , [10] , [11] , [12] . In terms of WAT, malfunction of mitochondrial activity can have a profound effect upon white adipocyte physiology [13] . Adipocyte mitochondria provide key intermediates for TG synthesis and are critical for lipogenesis; similarly, increased mitochondrial biogenesis is vital during the adipogenic process [14] , [15] . In addition, WAT mitochondria are pertinent for β-oxidation of liberated fatty acids during lipolysis, a key source of ATP to meet the energy demands during starvation [13] . Collectively, any mitochondrial disruption in adipocyte pathways contributes to the development of insulin resistance [13] , [14] , [16] , [17] . We previously generated a mouse model in which the amount of mitochondrial activity in adipocytes could be altered based on the properties of the outer mitochondrial membrane protein mitoNEET [18] . By overexpressing mitoNEET in adipocytes and combining the added metabolic challenge of a leptin-deficient ob/ob background, despite the prevalence of chronic obesity, mice exhibited system-wide improvements in insulin sensitivity; this provided a model of a ‘metabolically healthy’ obese state, with minimal lipotoxicity [18] . MitoNEET achieves these remarkable and potent effects on WAT expansion by modulating mitochondrial iron metabolism [18] . Here, to divert away from the severity of an ob/ob challenge and thus activation of secondary compensatory mechanisms, we examine the initial mechanisms by which mitoNEET triggers WAT expansion during HFD feeding. In particular, we identify that mitoNEET initiates a prominent transcriptional ‘browning’ programme during HFD exposure. The transgenic animals maintain the same weight as their wild-type littermates up to a point when this transcriptional browning programme fails to be maintained at a high level. At that point, WAT expandability capacity is enhanced in transgenic mice, prompting an immediate increase in body weight gain. Nevertheless, healthy WAT expansion prevails, with less HFD-driven inflammation and fibrosis evident with the local increase in mitoNEET, which ultimately results in an improved systemic metabolic profile. MitoNEET alters the browning signature of WAT Adipose-specific mitoNEET transgenic mice ( MitoN-Tg mice) undergo massive yet ‘healthy’ WAT expansion of the subcutaneous fat depot when metabolically challenged in a leptin-deficient ob/ob background [18] . While the ob/ob cross presents a severe metabolic challenge that rapidly elicits secondary compensatory mechanisms in WAT, we wanted to investigate mitoNEET action in a less-severe metabolic setting to establish the initial mitoNEET-induced effects that occur before massive WAT expansion. With this in mind, HFD feeding allows us to assess the gradual increase in body weight gain and potentially capture any key transcriptional or signalling events in which mitoNEET activates WAT expansion. Under chow-fed conditions, no marked differences in body weight gain were apparent between wild-type (WT) mice and MitoN-Tg mice ( Fig. 1a ). We subsequently challenged mice with a HFD (60% kcal fat). While no significant differences in body weight gain were evident during the initial 12 weeks of HFD feeding ( Fig. 1b ; arrow a), body weights reproducibly began to diverge around 13 weeks of HFD feeding, which gradually became more apparent by week 15 ( Fig. 1b ; arrow b). In light of this, we wanted to identify the critical determinants triggered by mitoNEET that initiate WAT expansion at this stage. We therefore performed microarray analyses on sWAT tissues specifically at week 12 of HFD feeding (before body weight divergence) and at week 15 of HFD feeding (post body weight divergence). 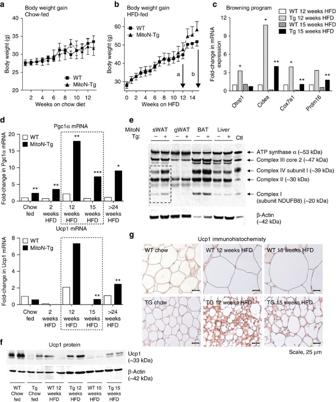Figure 1:MitoN-Tgmice exhibit increased body weight gain specifically at week 15 of HFD feeding due to a downregulation in the browning signature programme. Body weight gain in FVB wild-type (WT) mice and mitoNEET transgenic (MitoN-Tg) mice during (a) chow diet feeding or (b) high-fat diet (HFD) feeding. InFig. 1b, arrows a and b correspond to the 12- and 15-week stages of HFD feeding that microarray analysis was performed for, respectively. (c) Real-time qPCR confirmatory data of key BAT marker genes, reflective of a browning signature programme, identified from Illumina microarray profiling (Otop1,Cidea,Cox7a1andPrdm16) in sWAT derived from WT andMitoN-Tgmice fed HFD for either 12 or 15 weeks. Data represent fold change in gene expression when compared with WT sWAT under chow-fed conditions (n=5 per group). (d)Pgc1αandUcp1gene expression levels in WT sWAT andMitoN-TgsWAT derived from mice that were fed a chow-diet, or HFD for 2-, 12-, 15- or >24 weeks. Data represent fold change in gene expression when compared with WT sWAT under chow-fed conditions (n=5 per group). (e) Western blot of complex I (subunit NDUFB8), complex II, complex III (core 2), complex IV (subunit I) and ATP synthase α of the mitochondrial electron transport chain in WT and MitoN-Tg sWAT, gWAT, BAT and liver tissues (top panel). The lower panel shows β-actin expression levels. (f) Immunoblots showing Ucp1 protein expression (upper panel) and β-actin expression levels (lower panel), in addition to (g) Ucp1 immunohistochemistry (IHC) on WT sWAT andMitoN-TgsWAT from mice that were fed a chow diet, or HFD for 12 or 15 weeks (n=5 per group). All IHC images were obtained at × 40 magnification. Scale bar, 25 μm. Student’st-test, *P<0.05; **P<0.01; ***P<0.001. Table 1 highlights key genes markedly upregulated in MitoN-Tg sWAT between week 12 and week 15 of HFD feeding, which are either unaltered or oppositely regulated in WT sWAT during this timeframe; such genes include 11 β HSD1 , Erg1 , Sema5a , Col16a1 and Rarres2 (Chemerin). 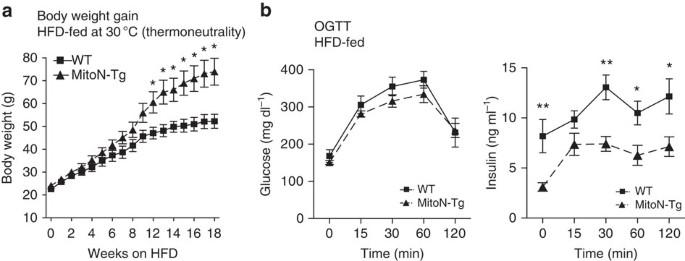Figure 2: Thermoneutrality promotes a faster rate of WAT expansion inMitoN-Tgduring HFD feeding. (a) Body weight gain in male FVB WT andMitoN-Tgmice during HFD feeding under thermoneutral conditions (~30 °C). (b) Glucose values (left) and insulin values (right) from an oral glucose tolerance test (OGTT) performed on WT versusMitoN-Tgfollowing 18 weeks of HFD feeding under thermoneutrality. Data represents mean±s.e.m. (n=7 per group). Student’st-test, *P<0.05; **P<0.01. Under similar conditions, Table 2 provides genes significantly downregulated between week 12 and week 15 of HFD feeding in MitoN-Tg sWAT. Interestingly, analysis revealed a marked reduction in the transcriptional signature programme that drives the ‘beiging’ phenotype of sWAT, with key brown adipose tissue (BAT) indicator genes including Otop1 , Cidea , Ucp1 , Cox7a1 and Cox8b ( Table 2 ). Figure 1: MitoN-Tg mice exhibit increased body weight gain specifically at week 15 of HFD feeding due to a downregulation in the browning signature programme. Body weight gain in FVB wild-type (WT) mice and mitoNEET transgenic ( MitoN-Tg ) mice during ( a ) chow diet feeding or ( b ) high-fat diet (HFD) feeding. In Fig. 1b , arrows a and b correspond to the 12- and 15-week stages of HFD feeding that microarray analysis was performed for, respectively. ( c ) Real-time qPCR confirmatory data of key BAT marker genes, reflective of a browning signature programme, identified from Illumina microarray profiling ( Otop1 , Cidea , Cox7a1 and Prdm16 ) in sWAT derived from WT and MitoN-Tg mice fed HFD for either 12 or 15 weeks. Data represent fold change in gene expression when compared with WT sWAT under chow-fed conditions ( n =5 per group). ( d ) Pgc1α and Ucp1 gene expression levels in WT sWAT and MitoN-Tg sWAT derived from mice that were fed a chow-diet, or HFD for 2-, 12-, 15- or >24 weeks. Data represent fold change in gene expression when compared with WT sWAT under chow-fed conditions ( n =5 per group). ( e ) Western blot of complex I (subunit NDUFB8), complex II, complex III (core 2), complex IV (subunit I) and ATP synthase α of the mitochondrial electron transport chain in WT and MitoN-Tg sWAT, gWAT, BAT and liver tissues (top panel). The lower panel shows β-actin expression levels. ( f ) Immunoblots showing Ucp1 protein expression (upper panel) and β-actin expression levels (lower panel), in addition to ( g ) Ucp1 immunohistochemistry (IHC) on WT sWAT and MitoN-Tg sWAT from mice that were fed a chow diet, or HFD for 12 or 15 weeks ( n =5 per group). All IHC images were obtained at × 40 magnification. Scale bar, 25 μm. Student’s t -test, * P <0.05; ** P <0.01; *** P <0.001. Full size image Table 1 Key microarray genes that are upregulated between 12–15 weeks HFD feeding. Full size table Table 2 Key microarray genes that are downregulated between 12–15 weeks HFD feeding. Full size table In addition, a reduction in mitochondrial β-oxidation pathways was evident; target genes downregulated at various steps of β-oxidation entailed Acadvl , Cyp2e1 , Cpt2 , Acaa2 , Slc25a20 , Aco2 , Decr1 and Etfb ( Table 2 ). With respect to browning, qPCR analyses confirmed the reduction in BAT-selective genes ( Otop1 , Cidea , Cox7a1 and Prdm16 ) between week-12 HFD versus week-15 HFD in MitoN-Tg sWAT ( Fig. 1c ). Surprisingly, when comparing WT sWAT versus MitoN-Tg sWAT at week 12 of HFD, a significant increase in factors mediating browning of WAT was apparent in mitoNEET transgenics ( Fig. 1c ). Of note, no marked differences in these browning genes were observed between WT sWAT and MitoN-Tg sWAT under chow-fed conditions ( Supplementary Fig. 1a ). To explore this browning aspect further, we examined the differential regulation pattern of two widely established BAT-indicator genes, Pgc1α and Ucp1 (refs 19 , 20 , 21 , 22 ). Under chow-fed conditions and 2 weeks of acute HFD feeding, Pgc1α message levels are significantly upregulated in MitoN-Tg sWAT ( Fig. 1d ). However, both Pgc1α and Ucp1 are profoundly upregulated in MitoN-Tg sWAT at 12 weeks of HFD feeding ( Fig. 1d ). In contrast, by week 15 of HFD, both Pgc1α and Ucp1 are significantly downregulated in transgenic sWAT; this downregulation persists even up to 24 weeks of HFD feeding ( Fig. 1d ). Consistent with the increase in Pgc1α expression under chow-fed conditions, we observed an upregulation in mitochondrial protein expression in MitoN-Tg sWAT, in particular complex I and complex IV of the mitochondrial electron transport chain (ETC) ( Fig. 1e ); such upregulation was specific for the subcutaneous fat pad, the primary site of mitoNEET overexpression. We previously reported that MitoN-Tg sWAT harbours mitochondria that are functionally compromised in oxidative respiration [18] . Here, the upregulation in mitochondrial protein is likely a Pgc1 α -dependent compensatory increase in mitochondrial biogenesis. The patterns of differential Pgc1 α and Ucp1 regulation in the transgenic sWAT were also evident at the protein level, as seen by western blot and immunohistochemical analyses ( Fig. 1f,g , respectively). Thermoneutrality enhances WAT expansion in MitoN-Tg mice The profound upregulation in the browning programme within MitoN-Tg sWAT during 12 weeks of HFD feeding ( Fig. 1c,d ) may serve as a key contributory factor that prevents full activation of WAT expansion in MitoN-Tg mice and therefore could partially explain the initial lack of difference in body weight gain between WT and MitoN-Tg mice up to 12 weeks of HFD feeding ( Fig. 1b ). To test this hypothesis, we metabolically challenged mice with HFD feeding under thermoneutral conditions, with the prediction that the euthermic conditions would minimize the effects of the large upregulation in browning in MitoN-Tg sWAT during the early stages of HFD feeding and thus a difference in body weight would become apparent within an earlier timeframe of HFD feeding. In particular, the thermoneutral zone in mice is ~30 °C. Such temperatures allow the lowest rate of energy expenditure required to maintain body temperature to be sustained [23] , [24] , [25] . Indeed, upon HFD feeding under thermoneutrality, MitoN-Tg mice gained significantly more body weight than WT mice, with body weight differences starting to diverge at the 8-week time-point already ( Fig. 2a ), indicating that MitoN-Tg mice display an earlier activation of WAT expansion through a reduction in the browning programme. Interestingly, despite MitoN-Tg mice displaying almost twice the size in body weight when compared with their WT littermates when kept under these thermoneutral conditions, thus receiving twice the glucose load, glucose clearance is fully preserved ( Fig. 2b ). This phenomenon is also observed in MitoN-Tg - ob/ob mice [18] . Figure 2: Thermoneutrality promotes a faster rate of WAT expansion in MitoN-Tg during HFD feeding. ( a ) Body weight gain in male FVB WT and MitoN-Tg mice during HFD feeding under thermoneutral conditions (~30 °C). ( b ) Glucose values (left) and insulin values (right) from an oral glucose tolerance test (OGTT) performed on WT versus MitoN-Tg following 18 weeks of HFD feeding under thermoneutrality. Data represents mean±s.e.m. ( n =7 per group). Student’s t -test, * P <0.05; ** P <0.01. Full size image In contrast to thermoneutrality, we performed cold tolerance tests to assess any potential defects in thermogenesis in MitoN-Tg mice either under chow-fed conditions or with HFD feeding. However, we noted no significant differences in body temperature between WT mice and MitoN-Tg mice either in an acute setting of cold exposure post chow-diet feeding, or a more chronic setting of cold exposure post HFD feeding ( Supplementary Fig. 1b ). MitoNEET-induced WAT expansion promotes insulin sensitivity To evaluate the extent to which mitoNEET impacts sWAT expansion, we sustained a more prolonged metabolic challenge of chronic HFD feeding. Interestingly, MitoN-Tg mice sustain almost twice the body weight in comparison to their WT littermates (WT: 48.3±1.3 g; MitoN-Tg : 82.0±2.0 g, Student’s t -test P <0.001) ( Fig. 3a ). Visually, micro-CT scans confirmed this gross AT expansion in MitoN-Tg mice following prolonged HFD feeding ( Fig. 3b ). Quantitatively, both sWAT and gWAT fat pads are significantly larger in adipose tissue (AT) volume ( Fig. 3c ), despite previously observing a marked reduction in gWAT fat pad size under chow-fed conditions [18] . 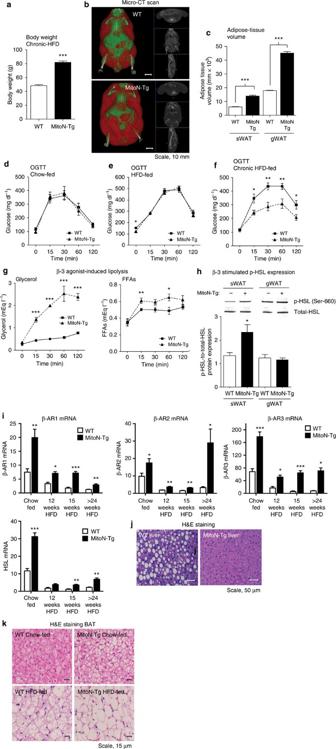Figure 3: During chronic HFD feeding,MitoN-Tgmice exhibit improved insulin sensitivity. (a) Body weights of WT mice andMitoN-Tgmice following chronic (>15 weeks) HFD feeding (n=5 per group). (b) A representative whole-body micro-CT scan of a chronic HFD-fed WT mouse (top) and a MitoN-Tg mouse (bottom). Scale bar, 10 mm. (c) sWAT and gWAT volume (mm × 103) (as determined by micro-CT scanning), following >15 weeks of chronic HFD feeding of WT mice andMitoN-Tgmice (n=5 per group). An oral glucose tolerance test (OGTT) (2.5 g kg−1body weight; single gavage) on FVB WT mice andMitoN-Tgmice following (d) chow-diet feeding, (e) 12 weeks of HFD feeding or, (f) chronic (>15 weeks) HFD feeding (n=5 per group). (g) Glycerol levels (left) and FFA levels (right) following a β-3 adrenergic agonist sensitivity test (1 mg kg−1CL316, 243 i.p., single injection;n=5 per group) of WT mice andMitoN-Tgmice that underwent chronic (>15 weeks) HFD feeding. (h) Representative immunoblots showing β-3 stimulated (1 mg kg−1CL316, 243 i.p., single injection) phospho-HSL (p-HSL) (Serine (Ser)-660) (top panel) and total-HSL (bottom panel) protein expression levels in WT andMitoN-TgsWAT and gWAT fat pads. Bar graphs show the calculated ratio of p-HSL-to-total-HSL protein expression levels in in WT andMitoN-TgsWAT and gWAT fat pads (n=4 per group). (i) Gene expression levels of β-adrenergic receptor 1 (β-AR1), β-AR2and β-AR3, in addition to hormone-sensitive lipase (HSL) in chow-fed, 12-week HFD-fed, 15-week HFD-fed and chronic (>24-week HFD-fed) WT versusMitoN-TgsWAT. Data represents mean±s.e.m. (n=5 per group). Student’st-test, *P<0.05; **P<0.01; ***P<0.001. (j) Representative H&E staining of chronic HFD-fed WT andMitoN-Tgliver tissues. All images were taken at × 20 magnification. Scale bar, 50 μm. (k) Representative H&E staining of BAT derived from WT mice andMitoN-Tgmice that were chow-fed (top panel) or chronic HFD-fed (bottom panel). Scale bar, 15 μm. Figure 3: During chronic HFD feeding, MitoN-Tg mice exhibit improved insulin sensitivity. ( a ) Body weights of WT mice and MitoN-Tg mice following chronic (>15 weeks) HFD feeding ( n =5 per group). ( b ) A representative whole-body micro-CT scan of a chronic HFD-fed WT mouse (top) and a MitoN-Tg mouse (bottom). Scale bar, 10 mm. ( c ) sWAT and gWAT volume (mm × 10 3 ) (as determined by micro-CT scanning), following >15 weeks of chronic HFD feeding of WT mice and MitoN-Tg mice ( n =5 per group). An oral glucose tolerance test (OGTT) (2.5 g kg −1 body weight; single gavage) on FVB WT mice and MitoN-Tg mice following ( d ) chow-diet feeding, ( e ) 12 weeks of HFD feeding or, ( f ) chronic (>15 weeks) HFD feeding ( n =5 per group). ( g ) Glycerol levels (left) and FFA levels (right) following a β-3 adrenergic agonist sensitivity test (1 mg kg −1 CL316, 243 i.p., single injection; n =5 per group) of WT mice and MitoN-Tg mice that underwent chronic (>15 weeks) HFD feeding. ( h ) Representative immunoblots showing β-3 stimulated (1 mg kg −1 CL316, 243 i.p., single injection) phospho-HSL (p-HSL) (Serine (Ser)-660) (top panel) and total-HSL (bottom panel) protein expression levels in WT and MitoN-Tg sWAT and gWAT fat pads. Bar graphs show the calculated ratio of p-HSL-to-total-HSL protein expression levels in in WT and MitoN-Tg sWAT and gWAT fat pads ( n =4 per group). ( i ) Gene expression levels of β-adrenergic receptor 1 (β -AR1 ), β -AR2 and β -AR3 , in addition to hormone-sensitive lipase (HSL) in chow-fed, 12-week HFD-fed, 15-week HFD-fed and chronic (>24-week HFD-fed) WT versus MitoN-Tg sWAT. Data represents mean±s.e.m. ( n =5 per group). Student’s t -test, * P <0.05; ** P <0.01; *** P <0.001. ( j ) Representative H&E staining of chronic HFD-fed WT and MitoN-Tg liver tissues. All images were taken at × 20 magnification. Scale bar, 50 μm. ( k ) Representative H&E staining of BAT derived from WT mice and MitoN-Tg mice that were chow-fed (top panel) or chronic HFD-fed (bottom panel). Scale bar, 15 μm. Full size image An initial evaluation revealed no significant differences in insulin sensitivity between WT mice and MitoN-Tg mice under chow-fed conditions ( Fig. 3d ), or upon exposure to a HFD challenge for up to 12 weeks ( Fig. 3e ; before the divergence in body weight gain ( Fig. 1b ; arrow a)). However, a significant difference in glucose tolerance only became apparent once MitoN-Tg mice were exposed to HFD following a period of more than 15 weeks. In particular, despite weighing more than their WT littermates, MitoN-Tg mice exhibit a marked improvement in glucose tolerance, even when glucose load is adjusted to total body weight ( Fig. 3f ); therefore, obese MitoN-Tg mice very effectively remove considerably more exogenous glucose from circulation than their WT littermates. In addition, chronic HFD-fed MitoN-Tg mice have the capacity to preserve their β-3 adrenergic agonist sensitivity. Following β-3 stimulation, MitoN-Tg mice exhibit significantly higher systemic levels of glycerol and FFAs ( Fig. 3g ). However, the FFA levels are vastly substoichiometric, an indication of substantial FFA re-esterification to TG, which is reflected by AT expansion. Hormone-sensitive lipase (HSL) is a key enzyme mediating the activation of lipolysis [26] . To further address the enhanced β-3 adrenergic agonist sensitivity in transgenic mice, we examined HSL phosphorylation following β-3 stimulation. A marked increase in phospho-HSL (p-HSL) was evident in MitoN-Tg sWAT, whereas no significant differences between MitoN-Tg gWAT and WT gWAT were apparent ( Fig. 3h ); the latter pinpoints the specificity of enhanced β-3 adrenergic agonist sensitivity to the mitoNEET-enriched sWAT. Gene expression analysis further corroborated an association between increased mitoNEET levels and β-3 adrenergic signalling pathways, as β-adrenergic receptor 1 (β -AR1 ), β -AR2 and β -AR3 , in addition to HSL expression levels were shown to be significantly upregulated in MitoN-Tg sWAT under chow-fed conditions. A similar upregulation was also observed in 12, 15 and >24-week HFD feeding studies ( Fig. 3i ). In line with improved whole-body insulin sensitivity in a state of chronic HFD feeding, histology further revealed minimal hepatic lipid accumulation in MitoN-Tg mice when compared with WT livers ( Fig. 3j ); collectively, accentuating that AT expansion minimizes obesity-induced hepatic steatosis and preserves insulin sensitivity. Finally, we previously reported some degree of mitoNEET overexpression was evident in BAT, albeit the subcutaneous fat pad predominantly harbours the bulk of mitoNEET overexpression [18] . We also noted that under chow-fed conditions, MitoN-Tg BAT is significantly larger in size when compared with WT BAT [18] . In light of this, we assessed BAT adipocyte size and observed that MitoN-Tg BAT harbours more lipid droplets under chow-fed conditions; moreover, HFD feeding appears to result in the formation of even larger adipocytes in MitoN-Tg BAT ( Fig. 3k ). Collectively, this suggests that while MitoN-Tg BAT is overall larger in size and harbours more lipid droplets under chow feeding, HFD feeding does not promote hyperplastic expansion in MitoN-Tg BAT, as typically observed in MitoN-Tg sWAT. MitoNEET favors M2 macrophage anti-inflammatory phenotypes Under chronic HFD-fed conditions, AT histology in MitoN-Tg sWAT appeared comparable to that of a healthy mouse on chow diet, with normal adipocyte cell size in comparison with enlarged hypertrophic adipocytes observed in WT sWAT under the same HFD conditions ( Fig. 4a ). To some extent, these differences were also preserved between WT gWAT and MitoN-Tg gWAT ( Fig. 4a ). Of note, we demonstrate that expression of the mitoNEET transgene is restricted primarily to adipocytes with minimal expression in other cell types, such as macrophages, with the highest level of mitoNEET expression observed in sWAT relative to gWAT and isolated macrophages ( Fig. 4b ; left). Moreover, we further assessed endogenous mitoNEET expression levels in adipocytes and the stromal vascular fraction (SVF) of both sWAT versus gWAT fat depots. We observed that the highest levels of mitoNEET are expressed in sWAT adipocytes, when compared with gWAT adipocytes ( Fig. 4b ; right). Furthermore, both sWAT and gWAT adipocyte fractions contained higher levels of mitoNEET relative to SVF derived from either sWAT or gWAT fat pads ( Fig. 4b ; right). Collectively, this demonstrates that endogenous mitoNEET levels are considerably higher in adipocytes than cells of the SVF (the latter containing cells such as preadipocytes, macrophages and endothelial cells); this may reflect the physiological roles that mitoNEET plays in each of these cell types. 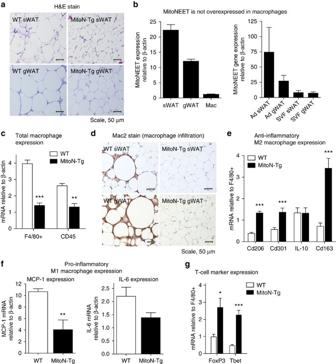Figure 4: MitoNEET promotes an M2 anti-inflammatory phenotype in sWAT. (a) Representative H&E staining of chronic (>15 weeks) HFD-fed WT andMitoN-TgsWAT (top panel) and gWAT (bottom panel). All images were obtained at × 20 magnification. Scale bar, 50 μm. (b) MitoNEET gene expression (relative to β-actin) in sWAT, gWAT and isolated macrophages (Mac) (n=5 per group) (left panel), in addition to adipocyte (Ad) fractions and SVF derived from unchallenged FVB WT andMitoN-TgsWAT and gWAT (right panel) (n=5 per group). (c) Total macrophage gene expression in WT andMitoN-TgsWAT following chronic HFD feeding (n=5 per group). (d) Representative images from Mac2 IHC staining of chronic HFD-fed WT andMitoN-TgsWAT and gWAT. All images were taken at × 20 magnification. Scale bar, 50 μm. (e) Anti-inflammatory M2 marker gene expression levels relative toF4/80+(Cd206,Cd301,IL-10andCd163) in chronic HFD-fed WT andMitoN-TgsWAT. Data represent mean±s.e.m. (n=5 per group). (f) Pro-inflammatory M1 marker gene expression levels, relative toF4/80+(Mcp-1andIL-6) in chronic HFD-fed WT andMitoN-TgsWAT (n=5 per group). (g) T-cell marker gene expression levels, relative toF4/80+(FoxP3andTbet) in chronic HFD-fed WT andMitoN-TgsWAT. Data represent mean±s.e.m. (n=5 per group). Student’st-test, *P<0.05; **P<0.01; ***P<0.001. Figure 4: MitoNEET promotes an M2 anti-inflammatory phenotype in sWAT. ( a ) Representative H&E staining of chronic (>15 weeks) HFD-fed WT and MitoN-Tg sWAT (top panel) and gWAT (bottom panel). All images were obtained at × 20 magnification. Scale bar, 50 μm. ( b ) MitoNEET gene expression (relative to β-actin) in sWAT, gWAT and isolated macrophages (Mac) ( n =5 per group) (left panel), in addition to adipocyte (Ad) fractions and SVF derived from unchallenged FVB WT and MitoN-Tg sWAT and gWAT (right panel) ( n =5 per group). ( c ) Total macrophage gene expression in WT and MitoN-Tg sWAT following chronic HFD feeding ( n =5 per group). ( d ) Representative images from Mac2 IHC staining of chronic HFD-fed WT and MitoN-Tg sWAT and gWAT. All images were taken at × 20 magnification. Scale bar, 50 μm. ( e ) Anti-inflammatory M2 marker gene expression levels relative to F4/80 + ( Cd206 , Cd301 , IL-10 and Cd163 ) in chronic HFD-fed WT and MitoN-Tg sWAT. Data represent mean±s.e.m. ( n =5 per group). ( f ) Pro-inflammatory M1 marker gene expression levels, relative to F4/80 + ( Mcp-1 and IL-6 ) in chronic HFD-fed WT and MitoN-Tg sWAT ( n =5 per group). ( g ) T-cell marker gene expression levels, relative to F4/80 + ( FoxP3 and Tbet ) in chronic HFD-fed WT and MitoN-Tg sWAT. Data represent mean±s.e.m. ( n =5 per group). Student’s t -test, * P <0.05; ** P <0.01; *** P <0.001. Full size image During HFD feeding, obesity initiates a state of low-grade inflammation and fibrosis, which ultimately pre-disposes to the progression to insulin resistance and T2DM [27] , [28] , [29] . In particular, obese AT harbours a high degree of infiltrating macrophages, typically termed AT macrophages (ФATMs); such ФATMs play an instrumental role in initiating a heightened state of chronic inflammation and associated metabolic dysfunctions [30] , [31] , [32] . More specifically, the type of ФATMs within AT contributes to the type of AT expansion during the progression of obesity. Several studies have demonstrated that ФATMs derived from lean mice express markers of M2 or ‘alternatively activated’ macrophages; conversely, obese states harbour a reduction in M2 markers, with concomitant increases in M1 or ‘classically activated’ macrophages [33] . Generally, an influx of M2 macrophages into AT is considered an anti-inflammatory characteristic that is associated with beneficial processes, such as angiogenesis and wound repair [33] . In contrast, M1 macrophage polarization is considered more pro-inflammatory and is associated with metabolic dysfunction and tissue destruction [33] . In light of this, we wanted to first establish whether mitoNEET-induced expansion of AT during HFD feeding promotes an influx of ФATMs and secondly if so, which type of macrophages infiltrate AT enriched with mitoNEET. Total macrophage marker gene expression levels, as determined by F4/80 + and Cd45 , were significantly lower in MitoN-Tg sWAT, when compared with WT sWAT ( Fig. 4c ). Consistent with this, Mac2 immunohistochemistry revealed considerably more macrophage staining in HFD-fed WT sWAT; displaying an increased presence of ‘crown-like’ structures (macrophages encircled around adipocytes) ( Fig. 4d ). In contrast, very few of these crown-like structures were observed in HFD-fed MitoN-Tg sWAT ( Fig. 4d ). Similarly, WT gWAT also harboured more macrophages and crown-like structures in comparison to MitoN-Tg gWAT ( Fig. 4d ). When examining the type of macrophages residing within HFD-induced obese AT, MitoN-Tg sWAT was shown to express significantly higher levels of the anti-inflammatory M2 macrophage markers Cd206 , Cd301 and Cd163 (when normalized to F4/80 + expression levels), in comparison to WT sWAT ( Fig. 4e ). Conversely, from a pro-inflammatory angle, MitoN-Tg sWAT was shown to express markedly less of the pro-inflammatory M1 macrophage markers MCP-1 and IL-6, when compared with WT sWAT ( Fig. 4f ). Finally, T cells have the capacity to infiltrate ‘inflamed’ obese AT and resolve some degree of inflammation [34] , [35] , [36] , [37] , [38] , [39] . In light of this, MitoN-Tg sWAT was shown to express significantly higher levels of the T-cell markers forkhead box P3 ( FoxP3 ) and the transcription factor T-bet (upon normalization to F4/80 + expression levels), when compared with WT sWAT ( Fig. 4g ). Previous studies have documented that WAT resident FoxP3-expressing regulatory T cells exhibit the capacity to reverse obesity-linked insulin resistance and decrease inflammation [40] , [41] . Moreover, mice deficient in the transcription factor responsible for the development of T helper cells, T-bet , while developing an obesogenic phenotype, exhibit hallmarks of an unhealthy metabolic profile [42] . Taken together, these studies suggest that during HFD-induced WAT expansion, MitoN-Tg sWAT harbours immune cells that promote an anti-inflammatory environment suitable for healthy WAT expansion. MitoNEET-driven healthy WAT expansion ameliorates fibrosis Given that we observe healthy AT expansion in MitoN-Tg sWAT following chronic HFD challenge, we subsequently assessed whether the overexpression of mitoNEET alters the vasculature. Gene expression profiling revealed that several endothelial markers are significantly upregulated in MitoN-Tg sWAT, when compared with WT sWAT, namely, Vegf , Vegf-R1 , Tie2 , Elastin , Cd31 and Flt-1 ( Fig. 5a ). Furthermore, trichrome staining of sWAT and gWAT fat pads revealed that HFD-challenged MitoN-Tg sWAT exhibits markedly less fibrosis in comparison to WT sWAT ( Fig. 5b ), again reflecting the healthy state of AT expansion under extreme metabolic challenges. Such differences in fibrotic WAT were further exacerbated in the gonadal fat pads between the WT and transgenic groups ( Fig. 5b ). We further observed significant decreases in Col3α1 and Col1α1 gene expression levels in HFD-fed MitoN-Tg sWAT, when compared with WT sWAT ( Fig. 5c ). Finally, we previously observed that gene expression markers of fatty acid (FA) uptake, adipogenesis and glucose uptake are upregulated in MitoN-Tg sWAT under chow-fed conditions [18] . Similarly, Fas , Fasn , Pparγ , Glut4 and Pepck gene expression levels were markedly increased in MitoN-Tg sWAT, when compared with WT sWAT ( Fig. 5d ). 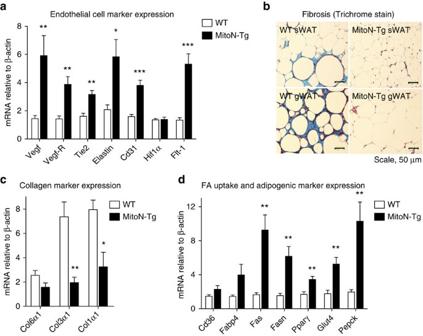Figure 5: MitoNEET promotes healthy WAT expansion during HFD feeding through stimulation of angiogenesis and reduction of collagens. (a) Endothelial cell marker gene expression levels relative to β-actin (Vegf,Vegf-R,Tie2,Elastin,Cd31,Hif1αandFlt-1) in chronic HFD-fed WT andMitoN-TgsWAT. Data represents mean±s.e.m. (n=5 per group). (b) Representative images of Trichrome-stained sWAT and gWAT derived from chronic HFD-fed WT mice andMitoN-Tgmice, reflecting the degree of WAT fibrosis. Scale bar, 50 μm. (c) Collagen marker gene expression levels relative to β-actin (Col6α1,Col3α1andCol1α1) in chronic HFD-fed WT andMitoN-TgsWAT (n=5 per group). (d) Fatty acid (FA) uptake, adipogenesis and glucose uptake marker gene expression levels relative to β-actin (Cd36,Fabp4,Fas,Fasn,Pparγ,Glut4andPepck) in chronic HFD-fed WT andMitoN-TgsWAT. Data represent mean±s.e.m. (n=5 per group). Student’st-test, *P<0.05; **P<0.01; ***P<0.001. Figure 5: MitoNEET promotes healthy WAT expansion during HFD feeding through stimulation of angiogenesis and reduction of collagens. ( a ) Endothelial cell marker gene expression levels relative to β-actin ( Vegf , Vegf-R , Tie2 , Elastin , Cd31 , Hif1α and Flt-1 ) in chronic HFD-fed WT and MitoN-Tg sWAT. Data represents mean±s.e.m. ( n =5 per group). ( b ) Representative images of Trichrome-stained sWAT and gWAT derived from chronic HFD-fed WT mice and MitoN-Tg mice, reflecting the degree of WAT fibrosis. Scale bar, 50 μm. ( c ) Collagen marker gene expression levels relative to β-actin ( Col6α1 , Col3α1 and Col1α1 ) in chronic HFD-fed WT and MitoN-Tg sWAT ( n =5 per group). ( d ) Fatty acid (FA) uptake, adipogenesis and glucose uptake marker gene expression levels relative to β-actin ( Cd36 , Fabp4 , Fas , Fasn , Ppar γ, Glut4 and Pepck ) in chronic HFD-fed WT and MitoN-Tg sWAT. Data represent mean±s.e.m. ( n =5 per group). Student’s t -test, * P <0.05; ** P <0.01; *** P <0.001. Full size image Adenoviral overexpression of mitoNEET promotes WAT expansion While the constitutive aP2 -driven transgene expression has proven to be a powerful tool to investigate the effects of mitoNEET overexpression, we subsequently intended to independently confirm our current findings. We therefore utilized an additional approach. To pinpoint the specificity and capacity of mitoNEET to expand AT during times of surplus caloric intake, we generated an adeno-associated virus carrying the mitoNEET cDNA (MitoN-AAV8) and hypothesized that upon viral delivery, a larger fat pad would emerge. To effectively infect adipocytes, we opted to utilize AAV serotype 8. We injected MitoN-AAV8 into the right sWAT fat pad of WT mice and, as an internal control we injected a control virus (Ctl-AAV8) into the left sWAT fat pad, which does not over-express mitoNEET ( Fig. 6a ). Both viruses contain a functional green fluorescent protein that allowed us to monitor the infection efficiency. Interestingly, the fat pad enriched with mitoNEET was markedly larger visually and in weight within 4 weeks post infection, despite both experimental and control fat pads being successfully infected with virus, as evident by the GFP signal ( Fig. 6b ). No apparent differences were observed for non-infected gWAT control fat pads ( Fig. 6b ). H&E staining of sWAT fat pads revealed no apparent differences in adipocyte size between Ctl-AAV8 sWAT and MitoN-AAV8 sWAT ( Fig. 6c ). Given that the MitoN-AAV8 fat pad is larger in size ( Fig. 6b ), and the average adipocyte size appears comparable, we conclude that an increase in adipogenesis is the likely explanation for the increase in fat pad size. This is overall consistent with the genetic mouse model of chronic overexpression. Finally, upon examination of WAT inflammation, we observed a significant reduction in gene expression levels of the pro-inflammatory marker TNF α in MitoN-AAV8 sWAT, when compared with Ctl-AAV8 sWAT, concomitant with a moderate increase in levels of the anti-inflammatory M2 macrophage marker, Cd163 expression ( Fig. 6d ). Collectively, this suggests that mitoNEET may further promote a non-inflamed environment for WAT expansion. 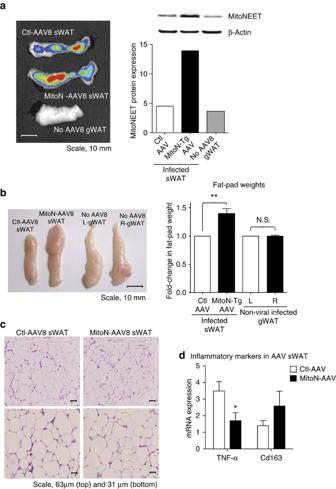Figure 6: Adenoviral-mediated overexpression of mitoNEET promotes AT expansion. (a) Epi-fluorescence scan (left panel) showing GFP signal (radiant efficiency ((p s−1cm−2sr−1) μW−1cm−2) (viral infection) and confirmation of mitoNEET protein overexpression in sWAT following viral injection (right panel). Scale bar, 10 mm. (b) A representative photograph (left panel) following direct injection of control virus (Ctl-AAV8-eGFP) or mitoNEET virus (MitoN-AAV8-IRES-eGFP) (5 × 1011PFU total sWAT injection) into left and right sWAT fat pads of 12-week-old WT FVB mice HFD-fed for 4 weeks, respectively. Scale bar, 10 mm. Non-infected left (L) and right (R) gWAT fat pads serve as additional internal controls. Fold change in L versus R sWAT (control or mitoNEET viral-infected, respectively) and L versus R gWAT (non-viral-infected) fat pad weights, following HFD feeding (4 weeks) of WT mice (right panel) (n=6 per group). Student’st-test, **P<0.01. (c) Representative H&E-stained images of Ctl-AAV8- (left) and MitoN-AAV8-infected (right) sWAT. Scale bar, 63 μm (top panel) and 31 μm (bottom panel). (d) TNFαand Cd163 gene expression levels in Ctl-AAV versus MitoN-AAV8 sWAT. Data represents mean±s.e.m. (n=4 per group). Student’st-test, *P<0.05. Figure 6: Adenoviral-mediated overexpression of mitoNEET promotes AT expansion. ( a ) Epi-fluorescence scan (left panel) showing GFP signal (radiant efficiency ((p s −1 cm −2 sr −1 ) μW −1 cm −2 ) (viral infection) and confirmation of mitoNEET protein overexpression in sWAT following viral injection (right panel). Scale bar, 10 mm. ( b ) A representative photograph (left panel) following direct injection of control virus (Ctl-AAV8-eGFP) or mitoNEET virus (MitoN-AAV8-IRES-eGFP) (5 × 10 11 PFU total sWAT injection) into left and right sWAT fat pads of 12-week-old WT FVB mice HFD-fed for 4 weeks, respectively. Scale bar, 10 mm. Non-infected left (L) and right (R) gWAT fat pads serve as additional internal controls. Fold change in L versus R sWAT (control or mitoNEET viral-infected, respectively) and L versus R gWAT (non-viral-infected) fat pad weights, following HFD feeding (4 weeks) of WT mice (right panel) ( n =6 per group). Student’s t -test, ** P <0.01. ( c ) Representative H&E-stained images of Ctl-AAV8- (left) and MitoN-AAV8-infected (right) sWAT. Scale bar, 63 μm (top panel) and 31 μm (bottom panel). ( d ) TNF α and Cd163 gene expression levels in Ctl-AAV versus MitoN-AAV8 sWAT. Data represents mean±s.e.m. ( n =4 per group). Student’s t -test, * P <0.05. Full size image Here, we have embarked on a detailed temporal analysis of the effects of mitoNEET overexpression in WAT. We find that upon exposure to HFD, mitoNEET as previously reported is likely to reduce the oxidative capacity of sWAT. However, as a compensatory mechanism, we observe that sWAT induces a significant ‘beiging’ programme that maintains the body weight of the transgenic animals. This compensatory increase is abruptly lost after ~12 weeks of HFD feeding, and it is at that time that weight differences start to become rapidly apparent. We can shift this period of weight gain by neutralizing the beiging effects of sWAT under thermoneutral conditions. During the expansion phase, minimal HFD-induced WAT inflammation prevails, with mitoNEET promoting anti-inflammatory M2 macrophages to reside within WAT, as opposed to pro-inflammatory M1 macrophages that typically reside within inflamed obese WAT. In addition, mitoNEET ameliorates HFD-driven fibrosis and promotes angiogenesis, the latter helping to sustain a fully vascularized fat pad during the expansion process. Collectively, abundant local mitoNEET levels in WAT result in profound improvements in whole-body systemic carbohydrate and lipid homeostasis, particularly with respect to preservation of insulin sensitivity, minimal obesity-induced hepatic steatosis and enhanced β-3 adrenergic agonist sensitivity. Finally, the mitoNEET-induced WAT expansion in vivo can be recapitulated using adenoviral-mediated injection of mitoNEET specifically into the subcutaneous fat pad, further pinpointing the primary mitoNEET-driven WAT expansion. White and brown adipocytes exert opposing functions in energy balance regulation [43] . White adipocytes store surplus energy in lipid droplets; conversely, brown adipocytes dissipate energy through non-shivering thermogenesis and may ameliorate diet-induced obesity through such an energy-wasting mechanism [23] , [44] , [45] . During the time spectra of HFD feeding, MitoN-Tg mice exhibit a unique differential pattern of beige AT-indicator gene expression during the progressive stages of sWAT expansion. In particular, Pgc1α and Ucp1 are vastly upregulated up to, and at, the 12-week stage of HFD feeding. Then, surprisingly by the 15-week stage of HFD feeding, both Pgc1α and Ucp1 are significantly downregulated in transgenic sWAT. We previously identified that an overexpression of mitoNEET in WAT compromises mitochondrial β-oxidation by lowering mitochondrial matrix iron content [18] ; such effects may result in insufficient iron–sulphur cluster import into the matrix, thus hindering mitochondrial respiratory complex formation and efficient electron transfer through the ETC. HFD-induced activation of the browning programme in transgenic mice at week 12 suggests a compensatory mechanism whereby mitochondria divert the excess energy from surplus dietary lipids away from an impaired ETC to utilize alternate avenues that enable energy dissipation as heat via Ucp1-dependent thermogenesis. Consistent with this notion, no difference in body weight is evident between WT mice and MitoN-Tg mice up to 12 weeks of HFD feeding; therefore, a vast upregulation in browning and thermogenesis could help cope with a large lipid influx into transgenic sWAT, as transgenics are known to exhibit an increase rate in lipid uptake [18] . Indeed, murine studies have demonstrated that overexpression of Ucp1 in WAT [15] and preadipocytes during adipocyte differentiation results in reduced accumulation of lipids [46] . Finally, the profound mitoNEET-induced downregulation in browning signature genes at week 15 HFD in transgenic sWAT likely activates unrestricted WAT expansion, which is mirrored by a divergence in body weight gain, with transgenic mice now displaying a marked increase in body weight gain. Thermoneutrality refers to the temperature at which the energy expenditure required to maintain body temperature is lowest [23] , [25] . Mice achieve thermoneutrality at ~30 °C. However, laboratory mice are typically housed at ‘room temperature’, generally 18 °C–22 °C and are therefore under chronic thermal stress and must increase their metabolism by ~50% (ref. 24 ). To potentially counteract the upregulation in browning events that occur before and up to the 12-week stage of HFD feeding that may hinder full activation of WAT expansion processes in MitoN-Tg mice, we applied the same metabolic challenge albeit under thermoneutral conditions. As expected, MitoN-Tg mice exhibit a steeper curve in body weight gain under thermoneutral conditions than under room temperature, as observed by body weight differences becoming apparent at 8-week HFD feeding, rather than at 15-week HFD feeding, respectively, thereby implicating earlier activation of WAT expansion mechanisms through a reduction in the browning programme. In fact under HFD-fed thermoneutral conditions, here we report the heaviest non- ob/ob mouse, which reached 114.2 g in body weight. Certainly, other studies have documented that during HFD feeding, Ucp1-deficient mice fail to become obese under laboratory conditions of 18 °C–22 °C (ref. 47 ), however become obese, although not remotely to the same degree as MitoN-Tg mice, when maintained under thermoneutrality [48] . Healthy WAT expansion has the capacity to prevent diet-induced lipotoxicity and the development of insulin resistance [5] . More specifically, each s.d. increase in sWAT mass decreases the chances of insulin resistance by 48%; conversely, each s.d. increase in visceral AT mass increases the chances of insulin resistance by 80% (ref. 49 ). MitoN-Tg mice undergo gross, yet hyperplastic sWAT expansion during chronic HFD feeding, which protects them from lipotoxicity and effectively preserves insulin sensitivity. Indeed, this metabolically healthy yet obese (MHO) paradox translates well to clinical findings, whereby unique subsets of morbidly obese patients are protected against obesity-related metabolic disturbances due to their capability to expand sWAT [50] , [51] , [52] . Despite a clinical awareness of MHO patients, which account for 20–30% of the obese population [52] , there is only a rudimentary understanding of factors and mechanisms underlying this phenotype and further underscores the need to identify and understand factors underlying the protective profile in MHO patients. Here, we identify a mouse model that mimics MHO patients, such that by altering the levels of a mitochondrial protein mitoNEET specifically in sWAT, we promote HFD-induced sWAT expansion and very effectively preserve carbohydrate homeostasis. With regards to examining mechanisms of sWAT expansion, our laboratory recently generated an inducible mouse model of permanently labelling mature adipocytes blue, which we coined the ‘AdipoChaser’ mouse [53] . Utilizing this unique mouse model, we identified that the majority of sWAT adipogenesis occurs early in life between embryonic days 14 and 18, and that later in life, with the addition of HFD feeding, sWAT expands through hypertrophic growth of adipocytes [53] . While in this current study we demonstrate that mitoNEET may promote HFD-induced hyperplastic sWAT expansion, as judged by smaller sWAT adipocytes upon metabolic challenge, future studies examining whether mitoNEET has the capacity to drive diet-induced adipogenesis in sWAT during the later stages in life, a phenomenon not typically observed in expanding sWAT, should prove illuminating. HFD-induced obesity is linked to a low-grade chronic pro-inflammatory state, in which macrophage infiltrate and reside within WAT and polarize from an anti-inflammatory M2 phenotype towards a pro-inflammatory M1 phenotype; this serves as a key contributory factor in the development of insulin resistance and T2DM [27] , [32] , [54] . Following HFD feeding, MitoN-Tg sWAT expresses high levels of the anti-inflammatory M2 macrophage markers and conversely, low levels of pro-inflammatory M1 macrophage markers, thereby collectively indicating that mitoNEET promotes healthy non-inflamed sWAT expansion. Consistently from a clinical perspective, Karelis et al. [50] noted that a favourable inflammation status was evident in the protective profile of obese MHO individuals. Angiogenesis is the process of new vasculature formation and is critical in providing growing and proliferating adipocytes with vascular supply during WAT expansion [29] , [55] ; a limited vascular source to expanding WAT can thus impede its maximal expandability capacity. The initiation of angiogenesis comprises the proliferation of endothelial cells and is mediated by the growth factor Vegf-A, acting through its receptor, Vegf-R2 (refs 56 , 57 ). HFD-induced expanding MitoN-Tg sWAT possesses a high maximal expandability limit, particularly under thermoneutrality, whereby we observe a 114.2 g non- ob/ob mouse. This is complemented with a significant increase in VEGF expression in MitoN-Tg sWAT, suggesting that proliferating adipocytes enriched with mitoNEET emanate angiogenic signals that trigger and ensure adequate vasculature formation and a robust blood supply that complements the rapidly expanding sWAT. Finally, in addition angiogenesis, for healthy sWAT to progress, the extracellular matrix (ECM) surrounding adipocytes, which principally consists of collagen, must be remodelled [29] . If ECM remodelling does not occur, an upregulation of ECM components occurs, at least in part as a response to the hypoxic conditions that prevail and lead to an upregulation of Hif1α, resulting in severe fibrosis [29] , [58] , [59] , a key feature in pathological sWAT expansion. Here, we observe that MitoN-Tg sWAT harbours markedly less HFD-induced fibrosis and lower collagen expression, thereby collectively confirming healthy, non-inflamed, non-fibrotic, highly vascularized models of sWAT expansion that ultimately preserve insulin sensitivity during HFD feeding. In summary, here we describe that during the initial stages of a HFD challenge, mitoNEET-enriched sWAT upregulates a browning programme that appears to dissipate surplus dietary energy for a period of up to 12 weeks. Shortly preceding this timeframe, mitoNEET then loses the ability to maintain this BAT programme in sWAT; this triggers WAT expansion, which is paralleled by sudden increase in body weight gain in the transgenic mice. It is not clear why the adipocytes lose their ability to maintain their BAT programme after 12 weeks on the HFD. This is driven by the number of weeks on the HFD, not by age of the mice. It is tempting to speculate that this may have something to do with the ‘crisis’ that occurs ~12–14 weeks into HFD feeding reported by Obin and colleagues [60] . This ‘crisis’ reflects widespread adipocyte death followed by re-emergence of new adipocytes that may differ in their differentiation programme and now no longer offer the compensatory upregulation of the BAT transcriptional programme. Animals All animal experimental protocols were approved by the Institutional Animal Care and Use Committee of University of Texas Southwestern Medical Center at Dallas. AT-specific mitoNEET transgenic mice were generated by subcloning the mitoNEET gene into a plasmid containing the 5.4-kb aP2 -promoter and a conventional 3′ untranslated region [61] . Following linearization, the construct was injected into FVB-derived blastocysts. Transgene-positive offspring were genotyped using PCR with the primer set: 5′-GGACCTCTGATCATCAAGA and 5′-GGAGACAATGGTTGTCAAC. All overexpression experiments were performed in a pure FVB background. All experiments were conducted using littermate-controlled male or female mice. All HFD experiments were initiated at ~6–12 weeks of age. Systemic tests and blood chemistry For the OGTT, mice were fasted for 3 h before administration of glucose (2.5 g kg −1 body weight by gastric gavage). At the indicated time-points, venous blood samples were collected in heparin-coated capillary tubes from the tail-vein. Glucose levels were measured using an oxidase-peroxidase assay (Sigma-Aldrich). Mice did not have access to food throughout the experiment. For the β 3 -adrenergic receptor-agonist sensitivity test, tail-vein serum samples were obtained before and 5-, 15- and 60 min following intraperitoneal injection of 1 mg kg −1 CL 316,243 (Sigma-Aldrich, St Louis, MO, USA). Insulin and adiponectin levels were measured using commercial ELISA kits (Millipore Linco Research, St Charles, MO). Glycerol and glucose levels were determined using a free glycerol reagent and an oxidase–peroxidase assay, respectively (Sigma-Aldrich). TG levels and cholesterol levels were measured using Infinity reagents (Thermo Fisher Scientific, Waltham, MA, USA). FFA levels were measured with a NEFA-HR(2) kit (Wako). Cold exposure For cold exposure experiments, ~12-week-old WT mice and MitoN-Tg mice were kept in individual cages and maintained on chow-diet for 3 d before cold exposure. During cold exposure, mice were fasted (4 h) before being housed in a cold cabinet (6 °C) with either no food (an acute setting of 6 h) or free access to food (chronic setting of 2 weeks HFD) and water. Computed topography For in vivo micro-CT scanning, mice were anaesthetized with 1% isoflurane inhalation and a whole-body scan was performed at a resolution of 93 μm (80 kV, 450 μA and 100 ms integration time) using an eXplore Locus Micro-CT scanner (GE Healthcare, Little Chalfont, Buckinghamshire, UK). The micro-CT scanner was calibrated according to protocols provided by the manufacturer. Each scan took ~10 min and the mice showed no sign of discomfort during the procedure. The images obtained were analysed using Microview software (GE Healthcare). Using the Microview software, WAT quantification was assessed from the base of the lungs to the distal side of the hip joint. For determination of total AT volume, histogram analysis of CT images showed that voxels with CT values between −380 and −120 Hounsfield units (HU) are defined as AT. The abdominal muscular wall was used as the differentiation line to separate sWAT from gWAT. Then, gWAT was analysed by assessing the fat content within the peritoneal cavity using the clearly visible peritoneum as guidance. The sWAT was obtained by subtracting gWAT from total body fat. Color-coded 3D-images of sWAT and gWAT were generated from the histograms using a volume-rendering tool (Microview software). Quantitative real-time PCR and microarray Tissues were excised from mice and snap-frozen in liquid nitrogen. Total RNA was isolated following tissue homogenization in Trizol (Invitrogen, Carlsbad, CA, USA) using a TissueLyser (Qiagen, Valenica, CA, USA), then isolated using an RNeasy RNA extraction kit (Qiagen). The quality and quantity of the RNA was determined by absorbance at 260/280 nm. cDNA was prepared by reverse transcribing 1 μg of RNA with SuperScript III reverse transcriptase and oligo(dT) 20 (Invitrogen). Table 3 highlights the primer sets that were used for quantitative RT–PCR. Results were calculated using the threshold cycle method [62] , with β-actin used for normalization. Table 3 Primer sequences. Full size table Immunoblotting Frozen tissue was homogenized using a TissueLyser (Qiagen) in TNET buffer (50 mM Tris–HCl (pH 7.6), 150 mM NaCl, 5 mM EDTA, phosphatase inhibitors (Sigma–Aldrich) and protease inhibitors [38] ), followed by low centrifugation and removal of any adipose layer present. Following addition of Triton X-100 to a final concentration of 1%, protein concentrations were determined using a bicinchoninic acid assay kit (Pierce). Proteins were resolved on either a 4–12% bis-Tris gel (Invitrogen) or a 10–20% Tricine gel (Invitrogen) and transferred to a polyvinylidene difluoride membrane (Millipore) or a nitrocellulose membrane (Protran, Whatman GmbH, Germany), respectively. A polyclonal antibody for Ucp1 was used (1: 250; Abcam, Cambridge, MA, USA). Polyclonal antibodies for total-HSL and p-HSL (Ser-660) were utilized (1:1,000; Cell Signaling Technology, Inc., MA, USA). A monoclonal MitoProfile Total OXPHOS Rodent Antibody Cocktail was also used (1:1,000; MitoSciences, Cambridge, MA, USA). Primary antibodies were detected using secondary immunoglobulin Gs labelled with infrared dyes emitting at 700 and 800 nm (1:5,000; Li-Cor Bioscience, Lincoln, NE, USA) and then visualized on a Li-Cor Odyssey infrared scanner (Li-Cor Bioscience). The scanned data were analysed using Odyssey Version 2.1 software (Li-Cor Bioscience). Full-length scans of immunoblots are shown in Supplementary Fig. 2 . Histology and immunohistochemistry The relevant fat pads or liver tissues were excised and fixed in 10% PBS-buffered formalin for 24 h. Following paraffin embedding and sectioning (5 μm), tissues were stained with H&E or a Masson’s Trichrome stain. For immunohistochemistry, paraffin-embedded sections were stained using polyclonal anti-Ucp1 antibodies (1:250; Abcam, Cambridge, MA, USA) or monoclonal anti-Mac2 antibodies (1:250; CEDARLANE Laboratories USA Inc., Burlington, NC, USA). AAV experiments WT mice were injected with Ctl-AAV8 or MitoN-AAV8 (5 × 10 11 PFU) (Vector Biolabs, PA, USA) directly into the left and right fat pads, respectively. Following HFD feeding (4 weeks), fat pads were monitored for GFP signal using a fluorescence scanner (IVIS, Caliper Life Sciences, MA, USA). Isolation of mouse peritoneal macrophages Peritoneal macrophages were collected from 12-week-old male FVB WT and MitoN-Tg mice by peritoneal lavage with 10 ml of PBS, centrifuged at 1,000 r.p.m. for 10 min and then resuspended in DMEM media supplemented with 10% fetal bovine serum. Cells were then incubated on a 24-well plate overnight before experimentation. Statistics All results are provided as means±s.e.m. All statistical analysis was performed using GraphPad Prism (San Diego, CA, USA). Differences between the two groups over time (indicated in the relevant figure legends) were determined by a two-way analysis of variance for repeated measures. For comparison between two independent groups, a Student’s t -test was utilized. Significance was accepted at a P value of <0.05. How to cite this article: Kusminski, C. M. et al. MitoNEET-mediated effects on browning of white adipose tissue. Nat. Commun. 5:3962 doi: 10.1038/ncomms4962 (2014).